Immunotoxin targeting glypican-3 regresses liver cancer via dual inhibition of Wnt signalling and protein synthesis Glypican-3 is a cell surface glycoprotein that associates with Wnt in liver cancer. We develop two antibodies targeting glypican-3, HN3 and YP7. The first antibody recognizes a functional epitope and inhibits Wnt signalling, whereas the second antibody recognizes a C-terminal epitope but does not inhibit Wnt signalling. Both are fused to a fragment of Pseudomonas exotoxin A (PE38) to create immunotoxins. Interestingly, the immunotoxin based on HN3 (HN3-PE38) has superior antitumor activity as compared with YP7 (YP7-PE38) both in vitro and in vivo . Intravenous administration of HN3-PE38 alone, or in combination with chemotherapy, induces regression of Hep3B and HepG2 liver tumour xenografts in mice. This study establishes glypican-3 as a promising candidate for immunotoxin-based liver cancer therapy. Our results demonstrate immunotoxin-induced tumour regression via dual mechanisms: inactivation of cancer signalling via the antibody and inhibition of protein synthesis via the toxin. Liver cancer is the fifth most common cancer worldwide [1] , [2] . According to the American Cancer Society ( www.cancer.org ), hepatocellular carcinoma (HCC) accounts for ~75% of all liver cancer cases. Despite the prevalence of HCC, surgery is still the most effective treatment to date but is only available for a limited number of patients identified at early stage [3] . For chemotherapy, sorafenib is the only-FDA-approved chemotherapeutic agent for HCC. It has only modest efficacy and most patients eventually develop resistance [4] , [5] . Therefore, there is an urgent need to develop new strategies for the treatment of liver cancers. Glypican-3 (GPC3) is a glycosylphosphatidylinositol (GPI)-anchored cell surface protein consisting of a core protein and two heparan sulfate (HS) chains [6] , [7] , [8] , [9] . GPC3 is highly expressed in 70–100% of HCCs but not in normal adult tissues [10] . Moreover, the expression of GPC3 is correlated with poor clinical prognosis in HCC [11] . GPC3 regulates many pathways in HCC pathogenesis, including Wnt [12] , [13] and Yap signalling [14] . GPC3 interacts with Wnt ligand and may function as a co-receptor for Wnt and facilitates Wnt/Frizzled binding for HCC growth [12] . Knocking down the expression of GPC3 in cell culture reduces Yap signalling [14] . Interestingly, soluble GPC3 protein (GPC3ΔGPI) can inhibit HCC cell growth. It may act as a dominant negative form to compete with endogenous GPC3, likely by neutralizing GPC3-binding molecules [15] , [16] . These studies confirm the proliferative effect of GPC3 in HCC and suggest that GPC3 is a potential target for HCC therapy. A humanized mouse monoclonal antibody (mAb; hGC33) that recognizes a C-terminal peptide of GPC3 inhibits tumour growth via antibody-dependent cellular cytotoxicity and is currently being evaluated in clinical trials [17] , [18] . To target GPC3, we generated three types of mAbs against GPC3: first, a mouse mAb (YP7) recognizing the C-terminal epitope that overlaps the hGC33-binding site [19] ; second, the human monoclonal antibody VH domain (HN3) targeting a conformational epitope in GPC3 that inhibits Yap signalling [14] ; third, we generated a human antibody (HS20) recognizing the HS chains on GPC3 that blocks Wnt signalling [13] . Although all of these antibodies show antitumor activity in vivo , none of them result in a regression of liver tumour growth when injected as naked antibodies. Immunotoxins are the chimeric proteins composed of an antibody fragment fused to a toxin. The variable fragment of the antibody directs the toxin to cancer cells that express an internalizing target antigen. We have used a 38-kDa truncated fragment of Pseudomonas exotoxin (PE38) to produce immunotoxins. PE38 contains the adenosine diphosphate-ribosylation domain that modifies elongation factor 2, leading to the arrest of protein synthesis and programmed cell death [20] . These types of toxins are very potent and are able to kill cancer cells resistant to standard chemotherapy, making them attractive agents against the cancers such as liver cancer, which are notorious for their multidrug resistance. We took advantage of the fact that GPC3 is highly expressed only on HCC cell surfaces to design antibody–toxin conjugates to enhance the efficacy of the ‘antibody alone’ strategy. The potency of an antibody–toxin conjugate depends on sufficient amounts of antigen on the cell surface and efficient internalization of target molecules. Among all the immunotoxins developed to date, CD22 immunotoxins are among the most effective for treating human cancer, in part, due to the rapid internalization of CD22 molecules from the surface of hairy cell leukaemia and other CD22-positive leukaemia cells [21] . The clinical success of immunotoxins also depends on the specificity of the drug to antigens expressed on cell surface [22] . In the present study, we find that GPC3 is efficiently internalized in HCC cells. We fuse HN3, the anti-GPC3 antibody that blocks Wnt signalling, to PE38 to construct a recombinant immunotoxin against GPC3. HN3-PE38 shows greater antitumour cytotoxicity than YP7-PE38 both in vitro and in vivo . Interestingly, the underlying mechanism of HN3-PE38 action involves inhibition of Wnt3a-induced β-catenin and Yap signalling. Intravenous administration of HN3-PE38 as a single agent or in combination with irinotecan induces regression of Hep3B and HepG2 tumours in mice. Our results demonstrate that GPC3 is a promising target for immunotoxins that act inside cells. We also show how the antibody portion of an immunotoxin not only determines tumour cell specificity but also enhances the cytotoxicity by blocking key signalling related to tumour growth. GPC3 is effectively internalized in HCC cells To explore whether GPC3 is a suitable target for immunotoxin, we investigated antigen density and internalization rates. First, we examined the expression levels of GPC3 on a panel of liver cancer cell lines. Three out of four GPC3-positive HCC cell lines have strong cell surface GPC3 staining ( Fig. 1a,b ; Supplementary Fig. 1 ). HepG2, a hepatoblastoma cell line, also had high protein expression of GPC3 on the cell surface. Huh-4 cells express an uncommon isoform of GPC3 that is not expressed on the cell surface. When we quantified the cell surface levels of G1 cells, which overexpress GPC3 in the A431 cell line, they had over 10 6 recombinant GPC3 sites per cell; all the cell lines expressing native GPC3 contain between 10 4 and 10 5 sites per cell ( Fig. 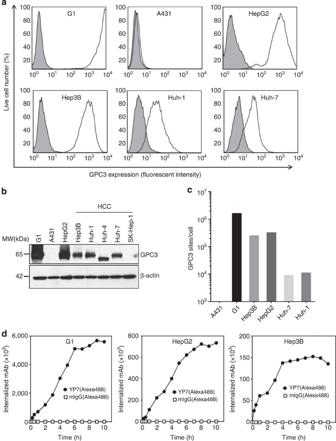Figure 1: GPC3 expression and internalization in HCC cells. (a) Flow cytometric results, detecting cell surface GPC3 expression in the GPC3-positive cell lines HepG2, Hep3B, Huh-1 and Huh-7. Cell line A431 does not express GPC3, and is shown as a negative control. G1 cells that overexpress GPC3 in the A431 cell line is shown as a positive control. Shaded grey peaks represent the cell surface staining with isotype control; white peaks represent the cell surface staining of GPC3. (b) Western blot analysis of endogenous GPC3 expression in HCC and other cell lines. For each sample, 20 μg total protein was loaded for detection. (c) Quantification of GPC3 sites per HCC cell using QuantiBrite PE beads. (d) Flow cytometric detection of internalization rates of GPC3. Each western blot and flow cytometric results representative of at least three independent experiments. MW, molecular weight. 1c ; Table 1 ). We chose to study Hep3B and HepG2, two widely used liver tumour models, in our study. Figure 1: GPC3 expression and internalization in HCC cells. ( a ) Flow cytometric results, detecting cell surface GPC3 expression in the GPC3-positive cell lines HepG2, Hep3B, Huh-1 and Huh-7. Cell line A431 does not express GPC3, and is shown as a negative control. G1 cells that overexpress GPC3 in the A431 cell line is shown as a positive control. Shaded grey peaks represent the cell surface staining with isotype control; white peaks represent the cell surface staining of GPC3. ( b ) Western blot analysis of endogenous GPC3 expression in HCC and other cell lines. For each sample, 20 μg total protein was loaded for detection. ( c ) Quantification of GPC3 sites per HCC cell using QuantiBrite PE beads. ( d ) Flow cytometric detection of internalization rates of GPC3. Each western blot and flow cytometric results representative of at least three independent experiments. MW, molecular weight. Full size image Table 1 GPC3 cell surface expression and internalization. Full size table Second, we investigated the internalization rate of GPC3 in HCC cells. An anti-GPC3 antibody, YP7 (ref. 19 ), was labelled with Alexa-488 and internalized fluorescence was measured by flow cytometry [22] . After 0.5 h, ~4 × 10 4 molecules were internalized by HepG2 and Hep3B cells and over 1 × 10 5 GPC3 molecules were internalized after 4 h ( Fig. 1d ; Table 1 ). Importantly, in all cell lines tested, we found that the amount of GPC3 internalized exceeded the amount bound on the cell surface by two- to fourfold, indicating that additional GPC3 molecules were recruited to the cell surface over time allowing more GPC3 internalization. Taken together, we found that GPC3 is highly expressed on the surface of HCC cells and is efficiently internalized by tumour cells. HN3-PE38 has superior cytotoxicity in vitro To test our hypothesis that GPC3 can be used as a therapeutic target of antibody–toxin conjugates in liver cancer, we constructed several immunotoxins using the antibodies recognizing different regions of GPC3 and a truncated form of PE38. All the immunotoxins were expressed in Escherichia coli , refolded in vitro and purified with satisfactory purity (>90%). The HS20 antibody binds a highly conserved epitope in the HS structure that is shared by other members of the glypican family, whereas the HN3 and YP7 antibodies specifically bind GPC3, not other glypicans ( Supplementary Fig. 2 ). Although GPC3 has been suggested as a promising target in liver cancer, it has not been clear whether other glypicans are also therapeutic targets in liver cancer or any other cancers. To choose highly selective agents for cancer therapy, we focused on immunotoxins derived from the HN3 and YP7 antibodies for further evaluation. We measured the binding affinities of HN3-PE38 and YP7-PE38 on purified GPC3 protein and cells expressing GPC3 on the surface. The binding affinity of HN3-PE38 was fourfold less than that of YP7-PE38 on GPC3 protein and over 20-fold less on tumour cells ( Fig. 2a ). 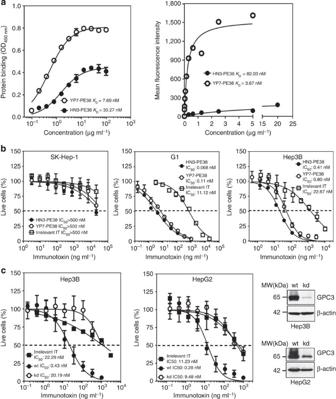Figure 2: Affinity and cytotoxicity of HN3-PE38 and YP7-PE38. (a) ELISA and flow cytometric analysis of HN3-PE38- and YP7–PE38-binding-affinities for GPC3 protein and G1 cells. The results are representative of at least three independent experiments. (b) Inhibition of cell proliferation on different cell lines by HN3-PE38 and YP7-PE38 immunotoxins, determined by a WST-8 assay. SK-Hep-1 was showed as an antigen-negative cell line. Dashed line indicated the value of IC50. IT, immunotoxin. Values represent mean±s.d. (c) Cytotoxicity of HN3-PE38 on wild type or GPC3 knocked down Hep3B and HepG2 cells. Western blot showed knockdown efficiency. wt, wide type; kd, knockdown. Dashed line indicated the value of IC50. Values represent mean±s.d. MW, molecular weight. Figure 2: Affinity and cytotoxicity of HN3-PE38 and YP7-PE38. ( a ) ELISA and flow cytometric analysis of HN3-PE38- and YP7–PE38-binding-affinities for GPC3 protein and G1 cells. The results are representative of at least three independent experiments. ( b ) Inhibition of cell proliferation on different cell lines by HN3-PE38 and YP7-PE38 immunotoxins, determined by a WST-8 assay. SK-Hep-1 was showed as an antigen-negative cell line. Dashed line indicated the value of IC 50 . IT, immunotoxin. Values represent mean±s.d. ( c ) Cytotoxicity of HN3-PE38 on wild type or GPC3 knocked down Hep3B and HepG2 cells. Western blot showed knockdown efficiency. wt, wide type; kd, knockdown. Dashed line indicated the value of IC 50 . Values represent mean±s.d. MW, molecular weight. Full size image To assess the cytotoxicity of HN3-PE38 and YP7-PE38, we examined the inhibition of cell proliferation on a panel of cell lines using the WST cell proliferation assay. Both HN3-PE38 and YP7-PE38 had high and specific cytotoxic activity against GPC3-positive cell lines but not GPC3-negative cell lines. Surprisingly, we found that HN3-PE38 was more effective than YP7-PE38 ( Fig. 2b ). On the basis of current knowledge, this observation was unexpected given that the efficacy of an immunotoxin is typically correlated with its antibody affinity [23] . To further evaluate the specificity of HN3-PE38, we evaluated the cytotoxicity of HN3-PE38 on GPC3 knockdown cells. When GPC3 expression in Hep3B cells and HepG2 cells was reduced, HN3-PE38 became less potent in growth inhibition assays, indicating the cytotoxicity of HN3-PE38 is dependent on GPC3 expression level ( Fig. 2c ; Supplementary Fig. 3 ). Overall, our data indicated that the HN3-PE38 immunotoxin potently inhibited liver tumour cell proliferation in vitro and had better antitumor activity than YP7-PE38. HN3-PE38 inhibits Wnt3a-induced signalling Since HN3-PE38 had significant lower affinity but was more efficacious than YP7-PE38, we hypothesized that the antibody portion of HN3-PE38 might enhance immunotoxin activity. To exclude the role of P. exotoxin , we introduced a point mutation (E553D) in its catalytic domain [24] and constructed two inactive immunotoxins: HN3-PE38 mut and YP7-PE38 mut. Compared with the original immunotoxins, mutant immunotoxins showed similar affinity on GPC3-expressing cells ( Fig. 3a ). We performed the [ 3 H] leucine incorporation assay to evaluate both active and inactive immunotoxins. The HN3-PE38 and YP7-PE38 inactive mutants did not inhibit protein synthesis, whereas the wild-type immunotoxins effectively inhibited protein synthesis ( Fig. 3b ). These results indicated that we successfully abolished the catalytic function of P. exotoxin without a significant change in the binding properties of the immunotoxins. We then compared the cytotoxicity of the inactive mutant immunotoxins: HN3-PE38 mut still retained a certain degree of cytotoxicity but YP7-PE38 mut was not active ( Fig. 3c ). This observation suggested that the HN3 antibody fragment may play an important role in the stronger cytotoxicity of the HN3-PE38 immunotoxin. 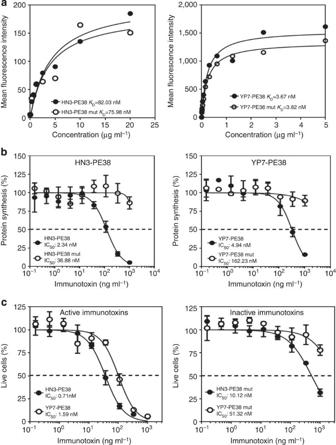Figure 3: Construction and analysis of inactive anti-GPC3 immunotoxins. (a) Flow cytometric analysis of active and inactive HN3-PE38- and YP7-PE38-binding affinities for G1 cells. TheKDvalues for G1 cells were based on mean fluorescence intensity (MFI). (b) [3H] Leucine incorporation assay to detect protein synthesis on Hep3B cells treated with active or inactive anti-GPC3 immunotoxins. Dashed line indicated the value of IC50. Values represent mean±s.d. (c) Cytotoxicity of active and inactive HN3-PE38 and YP7-PE38 on Hep3B cells, determined by a WST-8 assay. Dashed line indicated the value of IC50. Values represent mean±s.d. Figure 3: Construction and analysis of inactive anti-GPC3 immunotoxins. ( a ) Flow cytometric analysis of active and inactive HN3-PE38- and YP7-PE38-binding affinities for G1 cells. The K D values for G1 cells were based on mean fluorescence intensity (MFI). ( b ) [ 3 H] Leucine incorporation assay to detect protein synthesis on Hep3B cells treated with active or inactive anti-GPC3 immunotoxins. Dashed line indicated the value of IC 50 . Values represent mean±s.d. ( c ) Cytotoxicity of active and inactive HN3-PE38 and YP7-PE38 on Hep3B cells, determined by a WST-8 assay. Dashed line indicated the value of IC 50 . Values represent mean±s.d. Full size image It has been shown that GPC3 may promote Wnt/β-catenin signalling as a Wnt extracellular co-receptor [25] , [26] . The functional connection between GPC3 and Wnt signalling was also observed when we overexpressed GPC3 in HEK293 cells, stably expressing the Wnt reporter gene. The GPC3 overexpressing cells were more sensitive to Wnt ligand induction ( Supplementary Fig. 4 ). Our previous work showed that neutralizing the HS chains on GPC3 by a human antibody (HS20) blocked Wnt activation [13] . Interestingly, it has been reported that the protein core of GPC3 without HS also bound Wnt [12] , indicating that both the HS chains and the core protein of GPC3 may be involved in Wnt binding and activation and that targeting the GPC3 protein core by an antibody could also block Wnt signalling. To test our hypothesis, we analysed Wnt activation by treating HEK293 Topflash cells (which express endogenous GPC3) with enzymatically inactive immunotoxins against GPC3. We also made HS20-PE38 based on the HS20 antibody that reduced Wnt/β-catenin signalling via targeting the HS glycan chains on GPC3. As shown in Fig. 4a,b and Supplementary Fig. 5 , both HN3-PE38 mut and HS20-PE38 mut could inhibit Wnt/β-catenin signalling but YP7-PE38 mut had no effect. 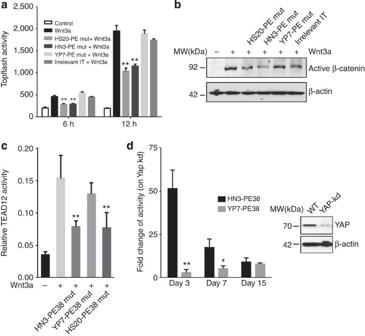Figure 4: Inhibition of Wnt3a-induced β-catenin and Yap signalling by inactive HN3-PE38. (a) Topflash activity of HEK293 Topflash cells treated with 0.5 μg ml−1inactive HN3-PE38 and YP7-PE38 in the presence of Wnt3a. Inactive HS20-PE38 and active irrelevant IT were set up as a positive and negative control, respectively. IT, immunotoxin. Values represent mean±s.d. **P<0.01 compared with Wnt3a-treated group, Student’st-test. (b) Active β-catenin expression on HEK293 Topflash cells treated as described inafor 12 h. (c) Yap/TEAD activity of Hep3B cells treated with 10 μg ml−1inactive HN3-PE38 and YP7-PE38 in the presence of Wnt3a for 16 h. Values represent mean±s.d. **P<0.01 compared with Wnt3a-treated group, Student’st-test. (d) Cytotoxicity of HN3-PE38 and YP7-PE38 on wild type and Yap knockdown Hep3B cells. Data were presented as fold change of IC50(wt versus kd). Western blot showed knockdown efficiency. Values represent mean±s.d., *P<0.05 and **P<0.01 compared with HN3-PE38-treated group, Student’st-test. wt, wide type; kd, knockdown; MW, molecular weight. Figure 4: Inhibition of Wnt3a-induced β-catenin and Yap signalling by inactive HN3-PE38. ( a ) Topflash activity of HEK293 Topflash cells treated with 0.5 μg ml −1 inactive HN3-PE38 and YP7-PE38 in the presence of Wnt3a. Inactive HS20-PE38 and active irrelevant IT were set up as a positive and negative control, respectively. IT, immunotoxin. Values represent mean±s.d. ** P <0.01 compared with Wnt3a-treated group, Student’s t -test. ( b ) Active β-catenin expression on HEK293 Topflash cells treated as described in a for 12 h. ( c ) Yap/TEAD activity of Hep3B cells treated with 10 μg ml −1 inactive HN3-PE38 and YP7-PE38 in the presence of Wnt3a for 16 h. Values represent mean±s.d. ** P <0.01 compared with Wnt3a-treated group, Student’s t -test. ( d ) Cytotoxicity of HN3-PE38 and YP7-PE38 on wild type and Yap knockdown Hep3B cells. Data were presented as fold change of IC 50 (wt versus kd). Western blot showed knockdown efficiency. Values represent mean±s.d., * P <0.05 and ** P <0.01 compared with HN3-PE38-treated group, Student’s t -test. wt, wide type; kd, knockdown; MW, molecular weight. Full size image HN3 inhibits HCC cell proliferation by blocking Yap signalling [14] . This inhibition may take place on the cell surface where HN3 binds to GPC3. However, the mechanism underlying how Yap signalling is triggered by cell surface molecules in mammals remains poorly understood. Interestingly, we found that Wnt3a could elevate Yap/TEAD reporter activity in Hep3B cells, suggesting that Wnt may be one of the cell surface regulators for Yap signalling ( Fig. 4c ). Unlike YP7-PE38 mut, HN3-PE38 mut significantly inhibited Wnt3a-induced Yap/TEAD signalling. In addition, Hep3B cells with Yap knockdown became remarkably more sensitive to HN3-PE38 than YP7-PE38 treatment: the half-maximal inhibitory concentration (IC 50 ) was 50-fold less than wild-type Hep3B cells, whereas YP7-PE38 only showed moderate difference (twofold less; Fig. 4d ; Supplementary Fig. 6 ). However, when Yap knockdown was stable (day 7 or later), the difference between HN3-PE38 and YP7-PE38 gradually disappeared. This observation suggested that Yap and GPC3 may cooperate with each other dynamically. Taken together, these data indicated that binding of HN3-PE38 to GPC3 on the cell surface inhibited both canonical Wnt/β-catenin signalling and Wnt3a-induced Yap signalling. HN3-PE38 exhibits potent antitumour activity in vivo To evaluate antitumour activity of HN3-PE38 and YP7-PE38 in vivo , we evaluated the toxicity in nude mice. We treated mice with four doses of HN3-PE38 and five doses of YP7-PE38 every other day for six injections. The mice tolerated 0.2, 0.4 and 0.8 mg kg −1 HN3-PE38 very well. However, the mice treated with YP7-PE38 immediately died after one injection at 0.4 and 0.5 mg kg −1 and two injections at 0.3 mg kg −1 , indicating YP7-PE38 was more toxic than HN3-PE38 ( Fig. 5a ). 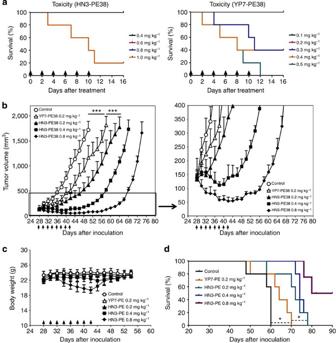Figure 5:In vivoantitumour activities of HN3-PE38 and YP7-PE38. (a) Toxicity detection of HN3-PE38 and YP7-PE38in vivo.BALB/c nu/nu mice were treated with indicated dose of immunotoxins intravenously every other day for a total of six injections. Arrow indicated individual injection;n=5/group. (b) Antitumour activity of HN3-PE38 and YP7-PE38. BALB/c nu/nu mice were s.c. inoculated with 5 × 106Hep3B cells. When tumours reached an average volume of 100 mm3, mice were administered indicated doses of immunotoxins intravenously every other day for six injections. Right panel showed amplified curves below 400 mm3. Arrow indicated individual injection;n=5/group. Values represent mean±s.e.m., ***P<0.001, paired Student’st-test. (c) Body weight of the mice treated inb. Arrow indicated individual injection;n=5/group. Values represent mean±s.e.m. (d) Survival curve for mice treated inb;n=5/group. *P<0.05, Log-rank (Mantel–Cox) test. Figure 5: In vivo antitumour activities of HN3-PE38 and YP7-PE38. ( a ) Toxicity detection of HN3-PE38 and YP7-PE38 in vivo. BALB/c nu/nu mice were treated with indicated dose of immunotoxins intravenously every other day for a total of six injections. Arrow indicated individual injection; n =5/group. ( b ) Antitumour activity of HN3-PE38 and YP7-PE38. BALB/c nu/nu mice were s.c. inoculated with 5 × 10 6 Hep3B cells. When tumours reached an average volume of 100 mm 3 , mice were administered indicated doses of immunotoxins intravenously every other day for six injections. Right panel showed amplified curves below 400 mm 3 . Arrow indicated individual injection; n =5/group. Values represent mean±s.e.m., *** P <0.001, paired Student’s t -test. ( c ) Body weight of the mice treated in b . Arrow indicated individual injection; n =5/group. Values represent mean±s.e.m. ( d ) Survival curve for mice treated in b ; n =5/group. * P <0.05, Log-rank (Mantel–Cox) test. Full size image To examine the antitumour activity of HN3-PE38 and YP7-PE38, we inoculated nude mice with Hep3B cells subcutaneously (s.c.). When the tumours reached an average volume of 120 mm 3 , the mice were treated with HN3-PE38 or YP7-PE38 intravenously every other day. At 0.2 mg kg −1 , the tumour size of the HN3-PE38-treated group was significantly smaller than the YP7-PE38-treated group. The antitumour activity of HN3-PE38 was dose-dependent: at 0.2 mg kg −1 , HN3-PE38 treatment delayed tumour growth; 0.4 mg kg −1 of HN3-PE38 stabilized tumour growth during the treatment. In the mice treated with 0.8 mg kg −1 of HN3-PE38, tumours showed regression; after we stopped the treatment, the tumours slowly grew back to the original size 16 days later ( Fig. 5b ). We also tested 0.4 mg kg −1 of YP7-PE38 on mice. However, all of the mice treated with 0.4 mg kg −1 of YP7-PE38 died, suggesting that it was impossible to evaluate YP7-PE38 at a high dose. The body weights of all the groups did not change significantly with the exception of the 0.8 mg kg −1 HN3-PE38-treated group. The body weight of this group decreased about 20% maximally during the treatment, but it rapidly returned to the normal level after we stopped the treatment ( Fig. 5c ). At a dose of 0.2 mg kg −1 , HN3-PE38-treated mice had significant survival extension as compared with YP7-PE38-treated mice; 0.4 mg kg −1 HN3-PE38-treated group did not seem to have significant benefits as compared with the 0.2 mg kg −1 group in overall survival. The 0.8 mg kg −1 group showed the best overall survival ( Fig. 5d ). We also performed immunohistochemistry staining on HN3-PE38- and YP7-PE38-treated tumours. HN3-PE38-treated tumours had less nuclear β-catenin and more phosphorylated Yap (p-Yap) staining, indicating the inactivation of canonical Wnt and Yap signalling by HN3-PE38 treatment in vivo ( Fig. 6 ). Together, HN3-PE38 had better antitumour activity than YP7-PE38 in mice. HN3-PE38 alone caused Hep3B tumour regression. 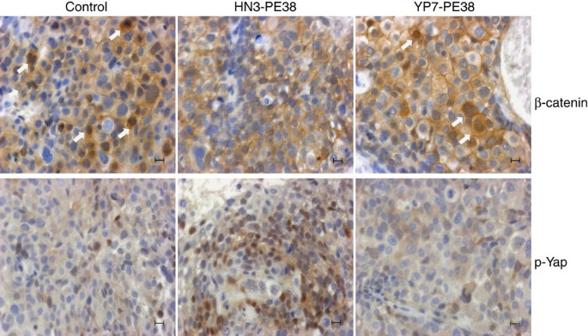Figure 6: Immunohistochemistry analysis of HN3-PE38- and YP7-PE38-treated tumours. β-Catenin staining and phosphorylated Yap staining on HN3-PE38- and YP7-PE38-treated Hep3B tumours. Scale bar, 50 μm. Arrow indicates nuclear staining of β-catenin. Figure 6: Immunohistochemistry analysis of HN3-PE38- and YP7-PE38-treated tumours. β-Catenin staining and phosphorylated Yap staining on HN3-PE38- and YP7-PE38-treated Hep3B tumours. Scale bar, 50 μm. Arrow indicates nuclear staining of β-catenin. Full size image Combining HN3-PE38 and chemotherapeutic therapies To enhance the therapeutic activity of immunotoxins in vivo , we also tested the combination treatment of HN3-PE38 with chemotherapeutic drugs. We initially combined HN3-PE38 with sorafenib, the approved drug in HCC, on the Hep3B xenograft model. However, the combination of sorafenib and HN3-PE38 did not show any improved antitumour activity ( Fig. 7a ). Therefore, we decided to test a panel of chemotherapeutic drug candidates that act through different mechanisms and that are approved or in clinical trials for treatment of different cancers [27] , [28] , [29] , [30] , [31] , [32] in HepG2 xenografts. Among them, irinotecan, a topoisomerase I inhibitor used to treat colorectal cancer [33] , showed the most potent antitumour activity ( Supplementary Fig. 7 ). We then combined HN3-PE38 with irinotecan in both the Hep3B model and the HepG2 model. HN3-PE38 was given intravenously every other day for a total of six injections, while irinotecan was given at a dose of 100 mg kg −1 intraperitoneally for just one injection before the immunotoxin treatment. The first injection of irinotecan was given 24 h before HN3-PE38 to allow sufficient time for irinotecan to damage endothelial cells and to allow for increased immunotoxin entry in the tumours [34] . In the Hep3B model, we used 0.4 mg kg −1 HN3-PE38 along with irinotecan to avoid body weight loss at 0.8 mg kg −1 . The combination of HN3-PE38 and irinotecan caused a modest tumour regression; once we stopped the treatment, tumours started to grow ( Fig. 7b ). In HepG2 model, HN3-PE38 alone was less effective. As a single agent, 0.6 mg kg −1 HN3-PE38 only delayed HepG2 tumour growth. This was probably due to the different cell context of HepG2 in which β-catenin is constitutively active [35] . In this case, the cytotoxicity of HN3-PE38 on HepG2 cells might only rely on the P. exotoxin part and not the antibody portion that could inhibit Wnt signalling. However, the combination of HN3-PE38 and irinotecan led to a synergistic tumour regression. The tumour size of this group quickly decreased to the detection limit (50 mm 3 ) only after one injection of HN3-PE38 and irinotecan ( Fig. 7c ). To further confirm the antitumour activity of the combination treatment of HN3-PE38 and irinotecan, we also measured the tumour weight and the serum alpha-fetoprotein (AFP) level, a liver cancer diagnosis marker, in mice after drug treatment. The serum AFP level was significantly reduced, correlating with the tumour shrinkage after treatment ( Fig. 7d–f ). 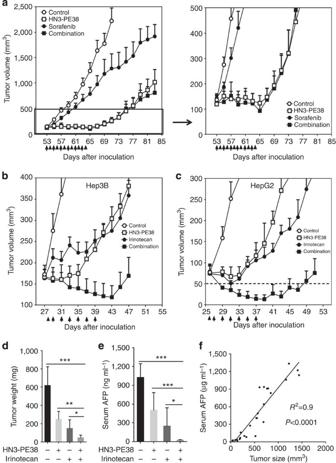Figure 7: Combination of HN3-PE38 immunotoxin with chemotherapeutic drugs. (a) Combination of HN3-PE38 with sorafenib on Hep3B model. BALB/c nu/nu mice with Hep3B tumour were treated with 100 mg kg−1sorafenib and 0.4 mg kg−1HN3-PE38 every other day for six injections when tumours reached an average volume of 120 mm3. Right panel showed amplified curves below 500 mm3. Arrow: HN3-PE38 injection; arrow head: sorafenib delivery;n=4/group. Values represent mean±s.e.m. (b) Combination of HN3-PE38 with irinotecan on Hep3B model. BALB/c nu/nu mice were treated with 100 mg kg−1irinotecan once and 0.4 mg kg−1HN3-PE38 every other day when tumours reached an average volume of 170 mm3. Arrow: HN3-PE38 injection; arrow head: irinotecan injection;n=5/group. Values represent mean±s.e.m. (c) Combination of HN3-PE38 with irinotecan on HepG2 model. BALB/c nu/nu mice were treated with 100 mg kg−1irinotecan once and 0.6 mg kg−1HN3-PE38 every other day for a total of six injections. Arrow: HN3-PE38 injection; arrow head: irinotecan injection;n=7/group. Values represent mean±s.e.m. Dashed line indicated the detection limit. (d) Tumour weight ofcon day 51. Values represent mean±s.e.m. *P<0.05, **P<0.01 and ***P<0.001, Student’st-test;n=7/group. (e) Serum AFP levels of the mice treated incon day 51. Values represent mean±s.d. *P<0.05, **P<0.01 and ***P<0.001, Student’st-test;n=7/group. (f) The correlation between AFP and tumour size. Correlation was measured by GraphPad Prism 6.0. Figure 7: Combination of HN3-PE38 immunotoxin with chemotherapeutic drugs. ( a ) Combination of HN3-PE38 with sorafenib on Hep3B model. BALB/c nu/nu mice with Hep3B tumour were treated with 100 mg kg −1 sorafenib and 0.4 mg kg −1 HN3-PE38 every other day for six injections when tumours reached an average volume of 120 mm 3 . Right panel showed amplified curves below 500 mm 3 . Arrow: HN3-PE38 injection; arrow head: sorafenib delivery; n =4/group. Values represent mean±s.e.m. ( b ) Combination of HN3-PE38 with irinotecan on Hep3B model. BALB/c nu/nu mice were treated with 100 mg kg −1 irinotecan once and 0.4 mg kg −1 HN3-PE38 every other day when tumours reached an average volume of 170 mm 3 . Arrow: HN3-PE38 injection; arrow head: irinotecan injection; n =5/group. Values represent mean±s.e.m. ( c ) Combination of HN3-PE38 with irinotecan on HepG2 model. BALB/c nu/nu mice were treated with 100 mg kg −1 irinotecan once and 0.6 mg kg −1 HN3-PE38 every other day for a total of six injections. Arrow: HN3-PE38 injection; arrow head: irinotecan injection; n =7/group. Values represent mean±s.e.m. Dashed line indicated the detection limit. ( d ) Tumour weight of c on day 51. Values represent mean±s.e.m. * P <0.05, ** P <0.01 and *** P <0.001, Student’s t -test; n =7/group. ( e ) Serum AFP levels of the mice treated in c on day 51. Values represent mean±s.d. * P <0.05, ** P <0.01 and *** P <0.001, Student’s t -test; n =7/group. ( f ) The correlation between AFP and tumour size. Correlation was measured by GraphPad Prism 6.0. Full size image Toxicology studies showed that this combination was well tolerated. All serum chemistry and blood cell counts in the group treated with HN3-PE38 and irinotecan were compared with the control group. All organ weights of the treated mice were statistically similar to the control group. HN3-PE38- and combination-treated groups had decreased serum albumin level. HN3-PE38-treated group also showed the decreased levels of haemoglobin and total serum protein; however, these parameters were restored when combined with irinotecan ( Table 2 ). These data demonstrate that the combinatory treatment of HN3-PE38 and irinotecan can significantly induce GPC3-positive tumour regression without any major side effects in vivo . Table 2 Toxicological results and organ weights. Full size table Here we described the new HN3-PE38 immunotoxin targeting GPC3, an oncofoetal antigen associated with Wnt molecules on the cell surface. The superior cytotoxicity of HN3-PE38 was based on the two mechanisms of action: inactivation of Wnt-induced signalling via the HN3 antibody portion and inhibition of protein synthesis via the bacterial toxin [20] . HN3-PE38 alone or in combination with irinotecan induced regression of liver tumour xenografts in mice. This study showed for the first time that an immunotoxin against GPC3 could be a potent strategy to achieve liver tumour regression. Although GPC3 is a cell surface biomarker highly expressed in HCC, the role of GPC3 in liver carcinogenesis remains elusive [14] , [18] . Currently, there are no GPC3 antibodies available that cause tumour regression. This highlights a major issue underlying the therapeutics of a naked GPC3 antibody that may not be potent enough for curative treatment of HCC. It would be reasonable to design immunotoxin to enhance the efficacy of the ‘antibody alone’ strategy. Furthermore, evidence suggests that GPC3 is involved in atypical multidrug resistance in cancer cells [36] . The cytotoxic effects of immunotoxins may bypass the signalling pathways related to multidrug resistance. There are a number of parameters that determine whether GPC3 will be an efficacious immunotoxin for treating HCC. First, the affinity of an antibody to its target is critical. We found that HN3-PE38 specifically bound the cell surface-associated GPC3 with a nanomolar K D . This affinity is sufficient to deliver toxin and inhibit tumour growth in vitro and in vivo . Second, the target antigen density on the cell surface may influence immunotoxin efficacy. With an average of 10 4 –10 5 , GPC3 molecules present on an HCC cell and the immunotoxin effect consequently correlates with GPC3 expression levels. This is consistent with previous observations regarding immunotoxins that target CD22-positive leukaemia cells [22] . Finally, the rate of internalization of a target antigen may be one of the most important parameters for any antibody–toxin conjugate that acts inside cells. Among all of the immunotoxins developed so far, anti-CD22 immunotoxins are among the most effective for treating human cancer, in part due to the fast and effective internalization of CD22 molecules [21] . HN3-PE38 internalizes efficiently with a similar rate to those of anti-CD22 molecules on leukaemia cells [22] . By achieving these criteria, HN3-PE38 shows promising cytotoxicity on GPC3-positive cells, inhibits HepG2 tumour growth and causes Hep3B tumour regression. In general, a major role of the antibody fragment is determining the cell specificity of immunotoxin. Immunotoxins with higher affinity normally bind more strongly, and for a longer time with the cell surface antigen, thereby exhibiting better efficacy [37] . In the present study, high-affinity immunotoxins do not improve killing efficiency once they reach a certain level (nanomolar K D value). More interestingly, an immunotoxin containing HN3 that blocks Wnt-induced signalling is more active than the one containing YP7 that has no effect on Wnt signalling. In regard to the generation of immunotoxins, our observation highlights the importance of choosing an antibody that blocks the signalling function of a cell surface receptor to achieve greater therapeutic value. In addition to the inhibition of canonical Wnt signalling, HN3-PE38 also blocks Wnt3a-induced Yap signalling. The expression of Yap has been shown to be regulated by β-catenin at the transcriptional level in colorectal carcinoma [38] . In the present study, inhibition of Wnt3a-induced Yap activity by HN3-PE38 may indicate that Yap is one of the target genes of canonical Wnt signalling. A recent study showed that Yap/TAZ is also involved in β-catenin destruction complex, releasing Yap/TAZ from the complex may initiate canonical Wnt signalling [39] . These results suggest that canonical Wnt and Yap signalling crosstalk through multiple mechanisms and might have feedback regulation in different cell contexts and tumour types. It was also interesting to note that Yap knockdown in Hep3B cells sensitized HN3-PE38 treatment in our cell proliferation assay. Our observations support potential crosstalk among Wnt, Yap and GPC3. We cannot rule out additional mechanisms that may involve the superior efficacy of HN3-PE38. Since HN3 only contains a VH domain, HN3-PE38 is smaller than YP7-PE38 (51 versus 64 KDa). This feature may cause a better tumour penetration of HN3-PE38 in vivo . In the present study, we found that both HS20-PE38 and HN3-PE38 inhibited Wnt/β-catenin and Wnt/Yap signalling. Although the HS20 antibody recognizes a conserved HS-related epitope and HN3 binds a unique epitope in the core protein of GPC3, our data indicates that both HS and the core protein of GPC3 are involved in Wnt/β-catenin and Wnt/Yap signalling activation. HN3-PE38 shows potent antitumour activity in Hep3B models. Even though HepG2 is a hepatoblastoma cell line, it has similar GPC3 expression and internalization rates. HN3-PE38 also inhibits HepG2 tumour growth, indicating HN3-PE38 may also be used to treat other GPC3-positive liver malignancies. Compared with Hep3B model, HN3-PE38 as a single treatment is less active in the HepG2 model. A possible explanation is that HepG2 cells express constitutively active β-catenin, and that HN3-PE38 may act only via toxin-mediated killing. On the other hand, HepG2 cells represent the heterogeneity of GPC3 expression in tumours. Our in vitro cell proliferation experiment shows that about 20% HepG2 cells were resistant to HN3-PE38 treatment and that this population was, in fact, GPC3-negative cells. Combination treatment of HN3-PE38 and irinotecan showed marked tumour regression in HepG2 tumours, but was less effective on Hep3B tumours. This phenomenon is consistent with reported clinical results: several phase II studies showed that irinotecan on HCC patients only had modest antitumour activity and significant adverse side effects [40] , [41] , [42] . However, another phase II study using irinotecan to treat refractory or recurrent hepatoblastoma in children has shown encouraging antitumour activity and acceptable toxicity [43] . HN3-PE38 alone or in combination with irinotecan shows tumour regression, thus supporting a novel approach for GPC3-positive liver malignancy therapy. We observed increased white blood cells in HN3-PE38 and the combination group, although statistically it was not different from the untreated group. Our previous study showed that mice treated with SS1P, an anti-mesothelin immunotoxin, did not increase white blood cell count [44] . Good manufacturing practice production will be needed for future comprehensive preclinical evaluation of HN3-PE38, including toxicity, pharmacokinetics, pharmacodynamics and biodistribution. In the present study, we used subcutaneous xenograft tumour models in mice as proof of concept to evaluate the antitumour efficacy of immunotoxins. Although subcutaneous xenograft tumour models are widely used to test therapeutic antibodies (including immunotoxins) for cancer therapy [37] , [31] , those models may not provide comparable tumour microenvironments as the primary tumour site. The limitations of xenograft models may not allow for further in-depth investigation on critical biological processes such as angiogenesis and metastasis [45] , [46] . It is expected that orthotopic models or other clinically relevant models may be more suitable for further validation of the efficacy of HN3-PE38 in liver cancer. Although immunogenicity induced by the bacterial toxin may limit the application of this strategy in humans, recent efforts have been made to attenuate immunogenicity. One promising approach appears to inhibit B- and T-cell activities [47] . Combination of the anti-mesothelin immunotoxin SS1P, together with immunosuppressant drugs, pentostatin and cyclophosphamide, which deplete T and B cells, achieved major tumour regression in mesothelioma patients [48] . It would be interesting to see whether similar combinatory approaches can be applied to liver cancer therapy with an anti-GPC3 immunotoxin. In conclusion, our results define a previously undescribed class of GPC3-targeted antibody–toxin chimeric molecules that are different from naked anti-GPC3 antibodies currently being evaluated in preclinical and clinical studies. Most importantly, this work unveils a biological rationale for targeting cell surface GPC3 with a functional antibody and its associated toxins. Our results also show the first example of how an antibody fragment of immunotoxin can enhance cytotoxicity by blocking major signalling in tumour cells. Furthermore, the anti-GPC3 immunotoxin alone or in combination with chemotherapy shows significant regression of human liver tumour xenografts in mice. The use of GPC3-targeted immunotoxins provides a new approach for treating liver cancer. Cell culture Six human HCC cell lines (SK-Hep-1, Hep3B, Huh-1, Huh-4 and Huh-7) were obtained from Xin-Wei Wang at the National Cancer Institute, Bethesda, MD, USA. SK-Hep-1 was originally isolated from a patient with adenocarcinoma of the liver but was redefined as a non-HCC line [49] . The HepG2 (hepatoblastoma) and A431 (epidermal carcinoma) cell lines were purchased from American Type Culture Collection (Manassas, VA, USA). G1 is a transfected A431 cell line stably expressing human GPC3. GPC3 knockdown cells and Yap knockdown cells were constructed by using gene-specific short hairpin RNA as described before [14] . HEK293 Topflash stable cell line was a kind gift from Dr Jeremy Nathans, Johns Hopkins Medical School. The cell lines were cultured in DMEM supplemented with 10% foetal bovine serum, 100 U ml −1 penicillin, 0.100 mg ml −1 streptomycin and 2 mmol l −1 L -glutamine. All cell lines were passaged <15 times. All cell lines were tested and authenticated by morphology and growth rate and were mycoplasma free. Flow cytometry Cells were trypsinized into single-cell suspensions and then incubated with 5 μg ml −1 YP7 or mouse IgG in FACS buffer (5% BSA and 0.01% NaN 3 ) for 1 h on ice. Bound antibodies were detected by incubating with a 1:200 dilution of goat anti-mouse IgG-PE secondary antibody (Invitrogen, Camarillo, CA, USA) in FACS buffer for half an hour on ice. For binding affinity measurement of immunotoxins, single-cell suspensions of A431-GPC3 cells were incubated with different concentrations of immunotoxins (starting with 10 μg ml −1 for YP7-PE38 and 20 μg ml −1 for HN3-PE38, 1:3 dilution) for 1 h on ice and then incubated with a 1:200 dilution of rabbit anti- P. exotoxin for 1 h on ice; bound antibodies were detected by goat anti-rabbit IgG-PE (Invitrogen) in FACS buffer for half an hour on ice. Cells were analysed using FACS Calibur (BD Biosciences, San Jose, CA, USA). The average number of GPC3 sites per cell was measured on a FACS Calibur (BD Biosciences) using BD Quantibrite PE beads (BD Biosciences) according to the manufacture’s instruction. For the time course of internalization, cells were incubated with 100 nmol l −1 Alexa-488-labelled YP7 at 37 °C for 0.25, 0.5, 1, 2 and 4 h. The cells were then stripped with glycine buffer 0.2 mol l −1 (pH 2.5) and 1mg ml −1 bovine serum albumin, to remove surface-bound Alexa-488-labelled YP7 and followed by analysis with FACS Calibur [22] . Western blotting Cells were lysed with radioimmunoprecipitation buffer (Cell Signaling Technology, Beverly, MA, USA) and the protein concentration was measured by Coomassie blue assay (Pierce Biotechnology, Rockford, IL, USA). Cell lysates (40 μg for each sample) were loaded into 4–20% SDS-PAGE gel for electrophoresis. The antibodies used included anti-GPC3 YP7 (ref. 19 ), anti-β-actin (Sigma, St Louis, MO, USA), anti-active β-catenin (Millipore, Temecula, CA, USA). Images have been cropped for presentation. Full-size images are presented in Supplementary Figures . Production of a recombinant immunotoxin As previously described in ref. 14 , the HN3 antibody was isolated on the full-length GPC3 protein from a human heavy-chain domain phage display library [50] . The YP7 antibody was isolated from mice immunized with a GPC3 peptide via hybridoma [19] . HN3 antibody VH domain, the YP7 antibody scFv fragment and the HS20 antibody scFv fragment were cloned into the NdeI and Hind-III restriction sites of the pRB98 vector [23] , [51] . The primer design and cloning procedure followed our standard protocol for immunotoxin production [52] . Two extra alanines were inserted between HN3 VH and PE38 as spacer. Cell proliferation inhibition assay Cells were seeded into 96-well plates at 10 4 per well. After overnight culturing, different concentrations of immunotoxins were added into wells. Cell growth inhibition was measured by WST-8 (Dojindo Molecular Technologies, Rockville, MD, USA) assays 48 h later. In some cases, the cells were pre-treated with immunotoxin for 30 min and then 50% Wnt3a conditioned media (CM) was added. The cytotoxicity was presented as IC 50 , which is the toxin concentration that reduced cell viability by 50% compared with the cells that were not treated with the toxin. Leucine incorporation assay Protein synthesis was measured by [ 3 H] leucine incorporation. The cells were seeded into 96-well plate at 10 4 per well. After overnight culturing, different concentrations of immunotoxins were added into wells. Sixteen hours later, the cells were pulsed with 1 μCi per well [ 3 H] leucine in 20 μl PBS, 0.2% human serum albumin for 2.5 h at 37 °C. The cells were frozen for 30 min at −80 °C, thawed for 1 h at 37 °C and processed in a harvester. Radiolabelled material was captured on filter mats and counted on a scintillation counter (GE Healthcare/Amersham Biosciences). Luciferase reporter assay HEK293 SuperTopflash cells were seeded into a 48-well plate. When the cells grew to 70% confluence, cells were treated with indicated concentrations of inactive immunotoxins. After 30 min, an equal volume of Wnt3a (CM) was added. Luciferase activity was measured and then normalized with total protein after 6 h and 12 h. For Yap reporter assay, Hep3B cells were seeded into 48-well plate. After overnight culturing, cells were transfected with 0.1 μg per well YAP/TEAD plasmid and 0.05 μg per well renilla luciferase plasmid. Twelve hours later, cells were pre-treated with inactive immunotoxins and Wnt3a CM as described above. Luciferase activity was detected 15 h later with the Dual-Luciferase Reporter Assay kit (Promega, Madison, WI, USA) according to the manufacturer’s protocol. Animal and tumour studies All mice were housed and treated under the protocol approved by the Institutional Animal Care and Use Committee at the National Institutes of Health (NIH). In most cases, 5 × 10 6 Hep3B cells or HepG2 cells were suspended in 200 μl of PBS and inoculated subcutaneously (s.c.) into 5-week-old female BALB/c nu/nu nude mice (NCI- Frederick Animal Production Area, Frederick, MD, USA). Tumour dimensions were determined using calipers and tumour volume (mm 3 ) was calculated by the formula V = ab 2 /2, where a and b represent tumour length and width, respectively. When the average tumour size reached ~100 mm 3 , the mice were intravenously injected with indicated dose of HN3-PE38 every other day. For combination with sorafenib, 3 × 10 6 Hep3B cells were s.c. inoculated into BALB/c nu/nu nude mice. Sorafenib (100 mg kg −1 ) was given to mice by oral delivery and HN3-PE38 treatment (0.4 mg kg −1 ) every other day for six injections. For combination of HN3-PE38 and irinotecan, one injection of irinotecan at 100 mg kg −1 was given to mice intraperitoneally one day before HN3-PE38 treatment; then followed by six injections of HN3-PE38 (intravenously, 0.4 mg kg −1 on Hep3B model and 0.6 mg kg −1 for HepG2 model). Mice were euthanized when the tumour size reached 1,000 mm 3 . For survival testing, mice were killed when tumour size reached over 3,000 mm 3 . Detection of serum levels of AFP Serum AFP levels were determined by enzyme-linked immunosorbent assay using an Enzyme Immunoassay kit (GenWay Biotech, Inc., San Diego, CA, USA). Whole-blood samples were collected from seven mice per group and on day 51 after the establishment of the xenograft. The concentration of AFP in the serum was measured according to the manufacturer’s instructions. The correlation between serum AFP and tumour size was calculated by GraphPad Prism 6.0 (San Diego, CA, USA). Toxicological analysis BALB/c nu/nu mice were s.c. inoculated with 5 × 10 6 HepG2 cells. When tumours reached an average volume of 100 mm 3 , mice were administered with HN3-PE38 (intravenously, every other day, 0.6 mg kg −1 for six injection), irinotecan (intraperitoneally, one injection before HN3-PE38 treatment, 100 mg kg −1 ) or both. Three mice from each group after drug testing were collected for toxicology studies. Samples were processed for completed blood counts, serum chemistry and organ weights and performed by Pathology/Histotechnology Laboratory in SAIC-Frederick. Statistical analysis All the representative results were repeated in at least three independent experiments. All group data (except those indicated) were expressed as the mean±s.d. of a representative experiment performed in at least triplicate and similar results were obtained in at least three independent experiments. All statistical analyses were conducted using GraphPad Prism 6.0. Differences between groups were analysed using the two-tailed Student’s t -test of means, with * P <0.05 defined as significant. How to cite this article: Gao, W. et al . Immunotoxin targeting glypican-3 regresses liver cancer via dual inhibition of Wnt signalling and protein synthesis. Nat. Commun. 6:6536 doi: 10.1038/ncomms7536 (2015).